Delayed commitment to evolutionary fate in antibiotic resistance fitness landscapes Predicting evolutionary paths to antibiotic resistance is key for understanding and controlling drug resistance. When considering a single final resistant genotype, epistatic contingencies among mutations restrict evolution to a small number of adaptive paths. Less attention has been given to multi-peak landscapes, and while specific peaks can be favoured, it is unknown whether and how early a commitment to final fate is made. Here we characterize a multi-peaked adaptive landscape for trimethoprim resistance by constructing all combinatorial alleles of seven resistance-conferring mutations in dihydrofolate reductase. We observe that epistatic interactions increase rather than decrease the accessibility of each peak; while they restrict the number of direct paths, they generate more indirect paths, where mutations are adaptively gained and later adaptively lost or changed. This enhanced accessibility allows evolution to proceed through many adaptive steps while delaying commitment to genotypic fate, hindering our ability to predict or control evolutionary outcomes. Antibiotic resistance can evolve through the sequential accumulation of multiple resistance-conferring mutations in a single gene [1] , [2] , [3] , [4] , [5] , [6] , [7] , [8] . Such multistep evolutionary pathways have been studied by reconstructing all possible intermediate genotypes between the ancestor and an evolved drug resistance genotype, to assess the feasibility of different pathways [9] , [10] . These studies show that only a limited number of pathways to the highly adapted genotype are feasible (continuously increasing in fitness), suggesting that epistatic interactions impose constraints that may render evolution more predictable [1] , [2] , [11] . However, adaptive landscapes can often have multiple distinct adaptive peaks, of which some may be more readily attainable than others [5] , [12] , [13] . Key to the predictability of evolution is whether and how early does evolution commit to a final genotypic state. By ‘commitment’ we refer to the idea that, as ongoing drug selection drives the sequential acquisition of resistance-conferring mutations, the number of resistant genotypic fates available to evolution is reduced and, out of the many initially available adaptive genotypic peaks, a single peak is finally chosen. Here we studied the evolutionary paths to trimethoprim resistance using a set of resistance-conferring mutations identified by laboratory evolution experiments, where five initially isogenic and drug-susceptible Escherichia coli populations were evolved in parallel under dynamically sustained trimethoprim selection, yielding several different drug-resistant genotypes [8] . These genotypes contained partially overlapping sets of mutations in the gene encoding trimethoprim’s target, dihydrofolate reductase ( DHFR ); each evolved strain had mutations in three out of five particular amino acids in DHFR and also a mutation in the DHFR promoter. We find that although genetic interactions limit the number of direct evolutionary paths to adaptive genotypes, where mutations are only gained, they greatly expand the number of indirect paths, where mutations can be adaptively lost or replaced by a different mutation at the same locus. This allows intermediate genotypes in the evolutionary process to trace feasible paths to many adaptive peaks, preventing early commitment to a genotypic fate. Furthermore, we find from simulations that this behaviour arises as a general property of multi-peak adaptive landscapes rich in high-order genetic interactions. Measurement of a multi-peaked adaptive landscape To map the adaptive landscape of trimethoprim resistance, we constructed and characterized all combinatorial sets of a collection of these resistance-conferring mutations [8] . We studied the effects of one promoter mutation (−35C>T, position relative to transcription start site) and five mutated amino acid residues, P21L, A26T, L28R, I94L and W30G/R, where at the W30 site we investigated two different types of mutations that were observed in the final genotypes ( Fig. 1a ). All possible combinations amounted to 96 DHFR variants (2 5 × 3 1 ), which were each synthesized and recombined into the E. coli chromosome in place of wild-type DHFR (Methods) [14] , [15] . Each strain was characterized in triplicate by measuring growth rates across a range of trimethoprim concentrations ( Fig. 1a , Supplementary Fig. 1 ). Briefly, a microtitre plate of the strain collection was inoculated into microtitre plates with liquid growth medium containing different trimethoprim concentrations. Plates were incubated at 30 °C with shaking, while optical density at 600 nm (OD 600 ) was measured every 45 min. Growth at each drug concentration was quantified as the definite integral of OD 600 from 0 to 30 h (this showed superior reproducibility to division rate; Supplementary Note 1 ). Drug resistance was quantified by IC75, the trimethoprim concentration that inhibits growth to 25% of wild-type drug-free growth ( Fig. 1b , Supplementary Data 1 , 2 ). IC75 measurements were highly reproducible across independent replicates, with experimental variance explaining <0.8% of the total variance in log(IC75) across the set of mutants ( Supplementary Fig. 2 ). 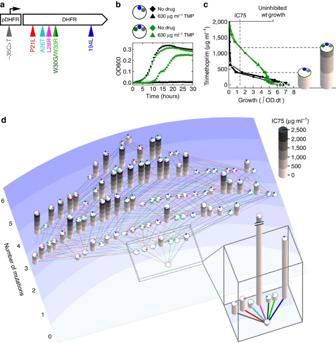Figure 1: Synthetic construction and phenotyping of all combinations of seven trimethoprim resistance mutations. (a) Trimethoprim (TMP) resistance can be conferred by any of seven different mutations in the target of trimethoprim,DHFR. Each combination of these mutations was synthesized and recombined into theE. coli DHFRgene. (b) The growth of each mutant strain was measured in liquid cultures spanning a range of trimethoprim concentrations, in triplicate. Growth is quantified by integrating optical density at 600 nm from 0 to 30 hours, and is illustrated by two strains, shown with no drug or with 630 μg ml−1trimethoprim. (c) Growth as a function of trimethoprim concentration is shown for the two example strains inb. The two drug concentrations shown inbappear here as diamond (no drug) and triangle (630 μg ml−1) markers. Trimethoprim IC75 is determined from this data as the drug concentration that inhibits growth to 25% of the wild-type growth without drug; three such independent measurements of each strain’s IC75 were performed. Each strain is represented by a column with height proportional to its IC75; atop each column are coloured circles that represent whichDHFRmutations are carried in that strain (colours matchinga). (d) The adaptive landscape of trimethoprim resistance conferred byDHFRmutations. Strains with differentDHFRmutations are distributed in rows sorted by number of mutations. Each gain of mutation throughout the network of genotypes is shown as a line coloured by the mutation gained. The trimethoprim resistance of the wild-type strain and each single mutant is shown with greater resolution in a vertically enlarged box. Figure 1: Synthetic construction and phenotyping of all combinations of seven trimethoprim resistance mutations. ( a ) Trimethoprim (TMP) resistance can be conferred by any of seven different mutations in the target of trimethoprim, DHFR . Each combination of these mutations was synthesized and recombined into the E. coli DHFR gene. ( b ) The growth of each mutant strain was measured in liquid cultures spanning a range of trimethoprim concentrations, in triplicate. Growth is quantified by integrating optical density at 600 nm from 0 to 30 hours, and is illustrated by two strains, shown with no drug or with 630 μg ml −1 trimethoprim. ( c ) Growth as a function of trimethoprim concentration is shown for the two example strains in b . The two drug concentrations shown in b appear here as diamond (no drug) and triangle (630 μg ml −1 ) markers. Trimethoprim IC75 is determined from this data as the drug concentration that inhibits growth to 25% of the wild-type growth without drug; three such independent measurements of each strain’s IC75 were performed. Each strain is represented by a column with height proportional to its IC75; atop each column are coloured circles that represent which DHFR mutations are carried in that strain (colours matching a ). ( d ) The adaptive landscape of trimethoprim resistance conferred by DHFR mutations. Strains with different DHFR mutations are distributed in rows sorted by number of mutations. Each gain of mutation throughout the network of genotypes is shown as a line coloured by the mutation gained. The trimethoprim resistance of the wild-type strain and each single mutant is shown with greater resolution in a vertically enlarged box. Full size image This network of genotypes and their associated IC75s produced a ‘rugged’ adaptive landscape with multiple peaks ( Fig. 1d ; Supplementary Note 2 for comparison with adaptive evolution study [8] ). Eleven of the 96 genotypes constitute ‘adaptive peaks’, where no gain or loss of a mutation is able to increase trimethoprim resistance ( Supplementary Fig. 3 ; some peaks are neutrally connected to others while others are fully separated by fitness valleys). An adaptive landscape can contain multiple peaks only if mutations’ phenotypic effects change sign (advantageous or deleterious) depending on the presence of other mutations, a genetic interaction called sign epistasis. (If mutations’ effects were positive on all backgrounds, there would have been a single adaptive peak containing all the mutations.) [16] , [17] Interestingly, while multiple peaks have previously been observed as the result of pairwise incompatibilities between mutations [7] , [18] , here every possible pair of mutated amino acids coexists in at least one adaptive peak ( Supplementary Fig. 3 ) suggesting a more complex origin for the observed ‘ruggedness’ than pairwise interactions. The landscape is shaped by high-order genetic interactions The fitness landscape has extensive high-order genetic interactions. A series of models of increasing complexity were constructed that described the log(IC75) of each genotype as a sum of parameters (equivalent to multiplying fold-changes in IC75) that represent the contributions to resistance of mutation’s effects alone and in pairwise or high-order combinations. A gradient of model complexity was created by finding which single parameter explained the most variance in IC75, then determining which second parameter contributed the next greatest increase in variance explained, and so forth ( Fig. 2a ). In this unbiased approach to detect explanatory effects and interactions, the promoter mutation (−35C>T) explained a large amount of variance because it more consistently provided a strong benefit, whereas the individual effects of amino acid mutations were overwhelmed by the genetic interactions that define their effects when present in various combinations ( Fig. 2b , Supplementary Fig. 4 ). For example, although L28R is by far the most beneficial mutation to acquire on the wild-type background, its effect is more context dependent when acquired on other backgrounds. To avoid ‘overfitting’ with spurious parameters, the Akaike Information Criterion [19] (AIC) was applied to assess the likelihood of each model relative to its number of parameters, revealing that over 60 genetic interaction terms, most of them high-order, made meaningful contributions to drug resistance ( Fig. 2a ). Pairwise genetic interactions reflect scenarios in which the effect of a mutation depends on the presence of another. Here we observed that, because of the multitude of high-order genetic interactions, the actual way in which two mutations interact varies based on the presence or absence of other mutations in the genetic background ( Fig. 2c , Supplementary Fig. 5 ). We next consider the effect of these genetic interactions on the adaptive paths and the commitment to evolutionary outcomes. 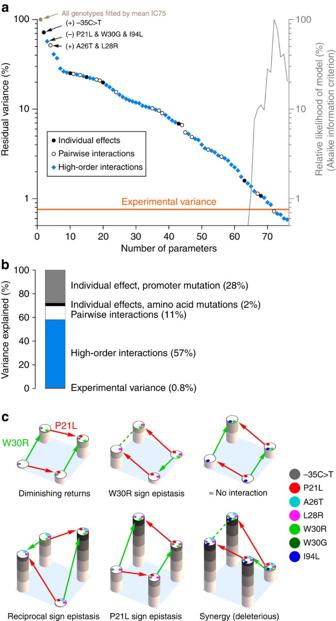Figure 2: High-order genetic interactions are prevalent in the adaptive landscape. (a) The log(IC75) of each genotype was fitted by a series of models of increasing complexity that assign changes in resistance through parameters that are based on the total number of mutations, the individual effects of mutations, and pairwise and high-order interactions between sets of mutations. 100% residual variance (0% variance explained) is defined by the sum of square errors in log(IC75) when every genotype is assigned the error-weighted mean IC75 (one parameter). Next the single parameter with the greatest explanatory power was chosen (a positive individual effect of the promoter mutation −35C>T), followed by the parameter with the second greatest explanatory power when combined with the first (a negative effect of P21L, W30G and I94L when all together), and so forth. Each point in the plot denotes the class of parameter added and the residual variance with that many parameters. The Akaike Information Criterion (AIC) was applied to determine the relative likelihood of each model, the most likely model being that which minimizes the AIC. (b) The variance explained by each category of parameter inawas summed (for example, all contributions of pairwise interactions). Only the promoter mutation (−35C>T) had a large individual effect, whereas the individual effects of amino acid mutations were small on account of strong genetic interactions. (c) The effect of many pairwise and high-order interactions is illustrated by viewing the qualitatively diverse effects and interactions of P21L (red) and W30R (green) when acquired on different genetic backgrounds. Mutations are indicated by coloured dots and column height represents trimethoprim resistance (IC75). Red (green) arrows indicate the favourable direction for gaining or losing the P21L (W30R) mutation. Genotypes with experimentally indistinguishable IC75 (no favoured direction) are connected by dashed lines.Supplementary Fig. 5shows the growth inhibition measurements of these strains. Figure 2: High-order genetic interactions are prevalent in the adaptive landscape. ( a ) The log(IC75) of each genotype was fitted by a series of models of increasing complexity that assign changes in resistance through parameters that are based on the total number of mutations, the individual effects of mutations, and pairwise and high-order interactions between sets of mutations. 100% residual variance (0% variance explained) is defined by the sum of square errors in log(IC75) when every genotype is assigned the error-weighted mean IC75 (one parameter). Next the single parameter with the greatest explanatory power was chosen (a positive individual effect of the promoter mutation −35C>T), followed by the parameter with the second greatest explanatory power when combined with the first (a negative effect of P21L, W30G and I94L when all together), and so forth. Each point in the plot denotes the class of parameter added and the residual variance with that many parameters. The Akaike Information Criterion (AIC) was applied to determine the relative likelihood of each model, the most likely model being that which minimizes the AIC. ( b ) The variance explained by each category of parameter in a was summed (for example, all contributions of pairwise interactions). Only the promoter mutation (−35C>T) had a large individual effect, whereas the individual effects of amino acid mutations were small on account of strong genetic interactions. ( c ) The effect of many pairwise and high-order interactions is illustrated by viewing the qualitatively diverse effects and interactions of P21L (red) and W30R (green) when acquired on different genetic backgrounds. Mutations are indicated by coloured dots and column height represents trimethoprim resistance (IC75). Red (green) arrows indicate the favourable direction for gaining or losing the P21L (W30R) mutation. Genotypes with experimentally indistinguishable IC75 (no favoured direction) are connected by dashed lines. Supplementary Fig. 5 shows the growth inhibition measurements of these strains. Full size image Hundreds of accessible evolutionary pathways Examining the accessible evolutionary trajectories, we found that adaptive mutation loss facilitated escape from seeming evolutionary ‘dead-ends’. Starting from the wild-type genotype we identified 483 adaptive trajectories where every step increases trimethoprim resistance (all continuously adaptive pathways were enumerated; Supplementary Fig. 6 presents methods to estimate pathway probabilities). Each trajectory ends at one of the ‘peak’ genotypes with strong and locally optimal trimethoprim resistance; it is an interesting feature, not necessarily universal, that no trajectories become trapped in local optima of modest trimethoprim resistance. Adaptation did not only proceed along ‘direct paths’, consisting only of gaining mutations. Instead, in many ‘indirect paths’, a mutation that was initially gained advantageously later became beneficial to lose due to interactions with newly gained mutations. Such adaptive mutational losses occur by converting to an alternative amino acid at the same site or by reverting to the wild-type amino acid ( Fig. 3a ). All but one of the amino acid mutations show some propensity for adaptive loss ( Fig. 3b ). At several genotypes, the only adaptive step within this finite landscape is mutational loss, indicating that without the consideration of mutation loss or the gain of different mutations to those studied here, it may appear – misleadingly – that trajectories could become stuck in evolutionary ‘dead-ends’ ( Supplementary Fig. 7 , example in Fig. 3a ). Thus, mutation reversion and conversion can contribute to evolvability on rugged adaptive landscapes, where some optima might otherwise be poorly accessible [9] . This property of the DHFR landscape is consistent with other empirically measured adaptive landscapes [2] , [5] , [20] . Mutational conversion and loss in DHFR was also directly observed in the forward evolution of trimethoprim resistance in E. coli , by daily genotyping of evolving populations [8] . It is unclear whether this tendency is particular to DHFR or if it may be common but is typically not observed when only initial and final evolved strains are genotyped. As the daily genotyping of evolving populations becomes increasingly practical, it will be interesting to test the generality of this property in different genes and environmental stresses. 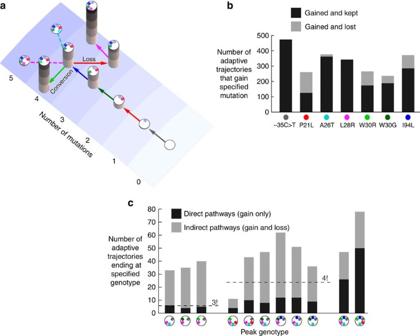Figure 3: Adaptive reversions and conversions bypass evolutionary dead-ends and expand the number of accessible evolutionary pathways. (a) Some evolutionary trajectories can only continue adaptation on this landscape through mutational reversion or conversion. In this example, after adaptively gaining four mutations, any further gain only lowers resistance, but a conversion or reversion can increase resistance. (b) Calculating all possible continuously improving trajectories over the adaptive landscape reveals that mutations are often gained but later adaptively lost. (c) The number of feasible evolutionary trajectories exceeds the maximum number possible without genetic interactions. All feasible trajectories are sorted by which of the adaptive peaks they reach, and coloured by whether they take a direct path in which mutations are only gained (black) or an indirect path in which some mutations may be gained and lost (grey). Dashed lines at 3! and 4! show the maximum possible number of direct pathways to genotypes with 3 or 4 mutations. When the number of pathways is belown!, genetic interactions constrain the number of pathways, and when aboven!, genetic interactions expand the number of pathways. Figure 3: Adaptive reversions and conversions bypass evolutionary dead-ends and expand the number of accessible evolutionary pathways. ( a ) Some evolutionary trajectories can only continue adaptation on this landscape through mutational reversion or conversion. In this example, after adaptively gaining four mutations, any further gain only lowers resistance, but a conversion or reversion can increase resistance. ( b ) Calculating all possible continuously improving trajectories over the adaptive landscape reveals that mutations are often gained but later adaptively lost. ( c ) The number of feasible evolutionary trajectories exceeds the maximum number possible without genetic interactions. All feasible trajectories are sorted by which of the adaptive peaks they reach, and coloured by whether they take a direct path in which mutations are only gained (black) or an indirect path in which some mutations may be gained and lost (grey). Dashed lines at 3! and 4! show the maximum possible number of direct pathways to genotypes with 3 or 4 mutations. When the number of pathways is below n !, genetic interactions constrain the number of pathways, and when above n !, genetic interactions expand the number of pathways. Full size image The process of mutational gain and subsequent loss generates indirect paths that greatly increase the number of evolutionary pathways leading to any specified peak. For each single-peak subset of the landscape with n mutations, there are n ! potential direct mutational paths leading to this peak (6, 24 or 120 paths to 3, 4 or 5 mutations, respectively). Consistent with previous studies of single-peaked adaptive landscapes [1] , [2] , [3] , many of these direct paths are restricted because genetic interactions render certain mutations deleterious on the background of other mutations ( Fig. 3c , black bars). However, considering all adaptive paths in the multi-peak landscape reveals many additional indirect paths in which gained mutations are subsequently adaptively lost or converted. These indirect paths are so abundant as to overcompensate for the reduction in direct pathways ( Fig. 3c , grey bars). Most indirect paths are only one or two steps longer than most direct paths ( Supplementary Fig. 8a ). Due to these indirect paths, the landscape has a higher level of connectivity; they increase the number of genotypes that can lead to any one peak ( Supplementary Fig. 8b ) and the number of peaks accessible from each genotype ( Supplementary Fig. 8c ). These properties are observed in this landscape, and not in previously characterized single-peaked landscapes, because it contains more mutations than only those in a single adaptive genotype. We thus anticipate that this increased accessibility due to indirect paths would only be more pronounced if a larger set of mutations was examined. Delayed commitment to evolutionary fate The increased accessibility of each adaptive peak in the actual landscape delays commitment to evolutionary fate much beyond what would be expected from simple models of adaptive landscapes. Landscapes without any sign epistasis contain only a single peak. Consider then a model adaptive landscape where pairwise epistasis creates multiple peaks: 2 k peaks can result from k incompatible pairs of mutations, where possessing any one member of the pair increases fitness but possessing both decreases fitness (that is, sign epistasis). In this simple model the number of peaks accessible to evolution halves with each adaptive mutation ( Fig. 4a ; similar results observed when multiple peaks are created by diminishing returns epistasis, Supplementary Fig. 9 ). In contrast to the simple theoretical landscape where the final genotype quickly becomes predictable, analysing all trajectories on the actual landscape reveals that they can proceed through many more steps with little reduction in the availability of different terminal fates ( Fig. 4a ; similar results obtained when applying this analysis to another experimental multi-peaked landscape [5] , Supplementary Fig. 10 ). This relaxed commitment is a direct result of the capacity for indirect paths; commitment is not delayed in the experimental landscape when mutational reversions and conversions are not permitted ( Supplementary Fig. 11 ). Indirect paths with delayed commitment to evolutionary fate appear in the measured adaptive landscape but not in the simple pairwise epistasis model. 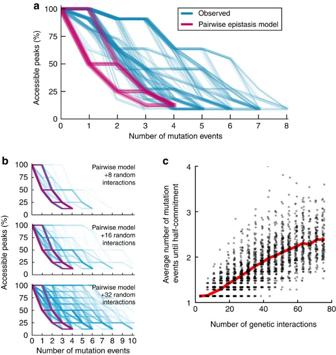Figure 4: High-order genetic interactions can delay commitment to evolutionary fate. (a) For each of the 483 adaptive pathways, the fraction of adaptive peaks that are potentially accessible from each genotypes along that path is plotted with respect to the number of mutational events (‘steps’) in a trajectory. Individual trajectories are shown with slight scatter in coordinates to visualize overlapping paths. Branching in the data reflects diversity amongst trajectories in the number of adaptive peaks that remain accessible. The observed properties of theDHFRlandscape (blue) are contrasted with a model of pairwise epistatic interactions (purple), where a peak is composed of an always beneficial promoter mutation plus any set of three binary choices between incompatible pairs of amino acid mutations (that is, choose one of mutationsaorb, choose one ofcord, and choose one ofeorf). (b,c) Beginning with the pairwise epistasis model (three second-order interactions, creating eight peaks), landscapes with a range of genetic interaction densities are created by adding interactions that are random in sign, magnitude and mutations involved (in groups of one each of second, third, fourth, and fifth order). Panelbshows how this addition of random genetic interactions (blue) postpones commitment to fate relative to the minimal pairwise model (purple), for ensembles of 100 such landscapes. The average number of mutations events until ‘half-commitment’—when half or fewer peaks remain accessible—is calculated for each landscape, with each trajectory weighted by its relative likelihood according to the equal fixation probability model1. Panelcshows how the number of mutations until reaching half-commitment is delayed with increasing numbers of random genetic interactions. Each dot is a landscape, and a red line follows the average of each ensemble of 200 simulated landscapes. Figure 4: High-order genetic interactions can delay commitment to evolutionary fate. ( a ) For each of the 483 adaptive pathways, the fraction of adaptive peaks that are potentially accessible from each genotypes along that path is plotted with respect to the number of mutational events (‘steps’) in a trajectory. Individual trajectories are shown with slight scatter in coordinates to visualize overlapping paths. Branching in the data reflects diversity amongst trajectories in the number of adaptive peaks that remain accessible. The observed properties of the DHFR landscape (blue) are contrasted with a model of pairwise epistatic interactions (purple), where a peak is composed of an always beneficial promoter mutation plus any set of three binary choices between incompatible pairs of amino acid mutations (that is, choose one of mutations a or b , choose one of c or d , and choose one of e or f ). ( b , c ) Beginning with the pairwise epistasis model (three second-order interactions, creating eight peaks), landscapes with a range of genetic interaction densities are created by adding interactions that are random in sign, magnitude and mutations involved (in groups of one each of second, third, fourth, and fifth order). Panel b shows how this addition of random genetic interactions (blue) postpones commitment to fate relative to the minimal pairwise model (purple), for ensembles of 100 such landscapes. The average number of mutations events until ‘half-commitment’—when half or fewer peaks remain accessible—is calculated for each landscape, with each trajectory weighted by its relative likelihood according to the equal fixation probability model [1] . Panel c shows how the number of mutations until reaching half-commitment is delayed with increasing numbers of random genetic interactions. Each dot is a landscape, and a red line follows the average of each ensemble of 200 simulated landscapes. Full size image Delayed commitment is created by high-order genetic interactions. Beginning with the aforementioned pairwise epistasis model, the progressive addition of random high-order genetic interactions (repeated over thousands of such landscapes) increases the number of evolutionary pathways and the average number of mutational steps taken until fate commitment ( Fig. 4b ; Supplementary Fig. 12 ). A simple model of three mutations suffices to illustrate how these effects occur. Second-order (pairwise) sign epistasis can generate two distinct peaks, but evolutionary paths on this landscape show fast commitment ( Fig. 5a ). However, adding a third-order interaction, whereby the sign epistasis of two mutations depends on the presence of the third (as often observed in the real landscape; Fig. 2c ), can maintain these two peaks while allowing indirect paths and postponing commitment to evolutionary fate ( Fig. 5b ). 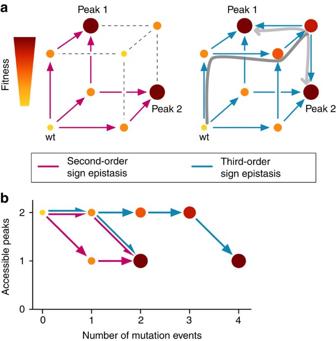Figure 5: A simple illustration of high-order epistasis causing delayed commitment. (a) The possible effects of high-order epistasis are illustrated by simple examples of multi-peaked landscapes consisting of three mutations. Circles represent genotypes, whose fitness is represented by circle size and colour. Arrows show the favored directions of evolutionary transitions; grey dotted lines mark transitions that cannot be realized. In these examples the mutation reached by a diagonal transition is always beneficial, while the mutations reached by horizontal and vertical transitions either always show reciprocal sign epistasis (second order), or only show reciprocal sign epistasis in the presence of the third mutation (third order). A grey line illustrates an indirect trajectory on the third-order landscape with late commitment. (b) The number of peaks accessible from each genotype inais plotted as a function of the number of mutation events in a trajectory. Second-order sign epistasis (purple) creates rapid commitment to fate: adaptive peaks are reached in at most two steps, and commitment can be made after a single step. Third-order sign epistasis (blue) creates longer trajectories with late commitment to fate: trajectories can take as long as four steps, and fate is never determined before a peak is reached. Figure 5: A simple illustration of high-order epistasis causing delayed commitment. ( a ) The possible effects of high-order epistasis are illustrated by simple examples of multi-peaked landscapes consisting of three mutations. Circles represent genotypes, whose fitness is represented by circle size and colour. Arrows show the favored directions of evolutionary transitions; grey dotted lines mark transitions that cannot be realized. In these examples the mutation reached by a diagonal transition is always beneficial, while the mutations reached by horizontal and vertical transitions either always show reciprocal sign epistasis (second order), or only show reciprocal sign epistasis in the presence of the third mutation (third order). A grey line illustrates an indirect trajectory on the third-order landscape with late commitment. ( b ) The number of peaks accessible from each genotype in a is plotted as a function of the number of mutation events in a trajectory. Second-order sign epistasis (purple) creates rapid commitment to fate: adaptive peaks are reached in at most two steps, and commitment can be made after a single step. Third-order sign epistasis (blue) creates longer trajectories with late commitment to fate: trajectories can take as long as four steps, and fate is never determined before a peak is reached. Full size image The evolution of trimethoprim resistance through mutations in the drug’s target DHFR is characterized by high-order genetic interactions that enable a multitude of indirect paths with mutational reversions and conversions. This abundance of feasible pathways increases the evolutionary accessibility of adaptive peaks, allowing the bypass of evolutionary dead-ends and postponing evolutionary commitment to fate. Simulations of adaptive landscapes showed that these effects crucially depend on, and are a general property of, high-order genetic interactions in adaptive landscapes. Therefore, more generally, when there exist multiple genotypic solutions to an evolutionary challenge, the net effect of genetic interactions is to increase the connectivity of the adaptive landscape and the number of feasible evolutionary pathways to any specified peak. This proliferation of adaptive paths on multi-peak landscapes considerably limits our ability to predict or control the course of evolution. The notion of an adaptive ‘end point’ is most relevant to the evolution of a specific functional change in a protein, such as drug resistance, but in the context of whole-genome evolution to a novel environment, adaptation may proceed for many thousands of generations [21] . Still a general principle emerges from this DHFR landscape that may apply also in this broader context: genetic interactions may strongly shape the course of evolution, but they do so as much by limiting opportunities as by presenting new ones. Strains and media All DHFR mutant strains were constructed in MG1655 attTn7::pRNA1-tdCherry (gift from N.D. Lord). Growth rate measurements were performed in a modified M9 minimal medium, for consistency with the forward evolution studies that identified the set of trimethoprim resistance mutations [8] (6 g l –1 Na 2 HPO 4 ·7H 2 O, 3 g l –1 KH 2 PO 4 , 5 g l –1 NaCl, supplemented with 0.4% glucose, 0.2% casamino acids and 1 mM MgSO 4 ). Drug solutions were made from powder stock (Sigma Aldrich: chloramphenicol, C0378; kanamycin, K1876; trimethoprim, T7883). Stock solutions of trimethoprim were prepared at 30 mg ml −1 in dimethylsulphoxide, and to avoid trimethoprim precipitation at high concentrations in media, working solutions were prepared by the slow addition of M9 media, with mixing, to the required volume of stock. Chromosomal integration Mutant DHFR strains were constructed by replacing the endogenous (coding and noncoding regions) of the DHFR gene with chemically synthesized mutant DHFR sequences, following the method of Datsenko et al . [14] specifically adapted for DHFR [15] . Briefly, mutant DHFR genes, including the native DHFR promoter, were synthesized and cloned into plasmid pKD13 that contained flanking kanamycin and chloramphenicol resistance genes. The integration cassette was PCR amplified with primers possessing 60 nucleotide homology to the genes immediately upstream ( kefC ) and downstream ( apaH ) of DHFR in the E. coli chromosome (upstream primer: 5′-GAAGAAGGTAAACATACCGGCAACATGGCGGATGAACCGGAAACGAAACCCTCATCCTAATCATGATCATCGCAGTACTGTTG-3′, downstream primer: 5′-AAGGCCGGATAAGACGCGACCGGCGTCGCATCCGGCGCTAGCCGTAAATTCTATACAAAACTGTCAAACATGAGAATTAATTC-3′; both PAGE purified). PCR products were DpnI digested (New England Biolabs, R0176) and electroporated into strains carrying the lambda Red recombinase expression plasmid pKD46 (ref. 14 ). Integrants were selected on lysogeny broth (LB) agar with 30 mg l –1 kanamycin and 25 mg l –1 chloramphenicol. Colony purification at 42 °C removed the pKD46 plasmid, which was confirmed by a failure to grow on LB agar with 100 mg l –1 ampicillin. Single colonies were Sanger sequenced to verify the sequence of the mutated DHFR locus. Gene synthesis services were provided by GenScript, oligonucleotide synthesis by Integrated DNA Technologies and DNA sequencing by GENEWIZ. Phenotyping assay Frozen stocks of all mutant strains were prepared in multiple master 96-well plates (M9 minimal media with 15% glycerol). For each replicate experiment, a frozen master plate was thawed and the contents diluted 33-fold into a deep 96-well plate of fresh M9 minimal media, to be used as an inoculation culture. A Liquidator 96 Manual Pipetting System (Mettler Toledo) was used to transfer 10 μl from each well of the inoculation culture plate into each of 29 experimental 96-well plates prepared with 140 μl of M9 minimal media and trimethoprim such that the final trimethoprim concentrations (after inoculation) spanned a 28-point range, from 0.16 to 3,400 μg ml –1 , with also duplicate trimethoprim-free plates. Plates were incubated with shaking in a ‘plate hotel’ (Liconic) in an environmental room at 30 °C and 70% humidity. Each well’s optical density at 600 nm (OD 600 ) was measured approximately every 45 min by an EnVision Multilabel Reader (Perkin Elmer). Growth and IC75 determination A background optical density of 0.03 units was subtracted from each OD 600 measurement, based upon the optical density of a control empty well present in all assays. A linear interpolation was created connecting measured data of OD 600 over time, which was then integrated over the time span from 0 to 30 h, giving a quantified measure of growth that is sensitive to drug-induced changes in growth rate as well as drug-induced changes in the duration of lag phase. Across the full set of over 2,500 growth measurements, 13 instances of aberrant growth were identified (0.5% of measurements), where growth of a particular strain at a particular trimethoprim dose was over twice the matching growth at the next lower trimethoprim concentration, and also twice the average growth of the other two replicates at the same trimethoprim concentration. These 13 aberrant measurements were substituted by the mean of their other two replicates. The trimethoprim resistance of each strain was quantified by the IC75, as calculated from the function of growth versus trimethoprim concentrations. Specifically, linear interpolations of growth versus log([trimethoprim]) were constructed, and IC75 was calculated as the largest trimethoprim concentration at which this linear interpolation of growth was equal to one quarter of the uninhibited wild-type growth. When simulating evolutionary trajectories ( Figs 3b and 4a ) and determining the directions of adaptive steps ( Fig. 2b ) we required 95% confidence that the IC75 values of neighbouring genotypes were not equal (based on the standard deviation of triplicate IC75 measurements), or else they were considered to be connected by neutral drift. Drift transitions between genotypes were not permitted in simulated evolutionary trajectories. Quantifying the complexity of genetic interactions A series of models were constructed to fit the trimethoprim resistance of each strain, as measured by log(IC75), using a series of terms that capture different ‘orders’ of mutational effects and genetic interactions. The presence or absence in a strain of each mutation i is referred to by terms m i that equal 0 when that mutation is absent or 1 when present ( i ranges from 1 to 7 for the 7 different mutations characterized). The contribution of each individual mutation i to log(IC75) was described by the terms c i . The effect on log(IC75) of possessing the pair of mutations i and j (two-way interaction) was described by the term c i,j . Similarly, three-way interactions were described by terms c i,j,k , four-way interactions by c i,j,k,l and five-way interactions by c i,j,k,l,n . In the most complex model that includes all terms up to five-way interactions, the log(IC75) of each strain is thus described by: Parameter fitting was performed by minimizing the term: using the Minimize function of Mathematica 9.0. Error in log(IC75 observed ) was estimated when analysing growth inhibition measurements (see ‘Growth rate and IC75 determination’ above), and here is taken to be the larger of either the estimated experimental error or the concentration step between experimentally utilized trimethoprim concentrations ( Supplementary Fig. 1 ). For example, if IC75 was estimated as 1,200 μg ml −1 , being between experimental measurements of growth at 1,000 and 1,400 μg ml −1 trimethoprim, error in log(IC75) is at least log(1,400)–log(1,000). The seven particular combinations of mutations that could not be engineered into the E. coli chromosome, plus one strain with <25% of wild-type growth even in the absence of drug, were not included when summing the error over strains. 100% of variance was defined as this error term when IC75 fitted was equal to the mean IC75 of all measured strains. A gradient of model complexity was created by first testing all single parameters and identifying the one parameter that produced the best fit (that is, explained the most variance). Next, all remaining parameters were tested together with the first chosen parameter to identify which two parameters produced the best fit. In this subsequent fit, the numerical value of first selected parameter was allowed to change to reflect the new discrimination amongst genotypes introduced by the second parameters. This process was iterated, adding one parameter each round. The AIC of each model was calculated as 2. k –2.log( L ), where ‘ k ’ is the number of parameters in the model and ‘ L ’ is the likelihood of measuring the observed IC75 values if the true values were those predicted by the model [19] . Specifically, the likelihood of a model was the product of the likelihoods of each strain’s IC75 measurement. The likelihood that a given IC75 measurement would be made for strain i is the probability density at the observed log 10 (IC75) (observation i ) of a normal distribution centred on the predicted log 10 (IC75) (prediction i ) with standard deviation equal to the larger of either the estimated experimental error or the concentration step between experimentally utilized trimethoprim concentrations (error i ). Mathematically, model likelihood L is: where the denominator serves to normalize probability density in the elements of the product: The model with the greatest relative likelihood is considered to be that with the minimum AIC value (AIC min , which was the model with 72 parameters). The relative likelihood of all other models i was calculated by Exp((AIC min –AIC i )/2) (ref. 19 ). Simulating landscapes with randomized genetic interactions A model adaptive landscape was constructed that was similar in composition to the observed trimethoprim-resistance landscape except containing, initially, only second-order genetic interactions. Thus, seven mutations were defined each with fitness effect +1, where one mutation was always beneficial (approximating the −35C>T promoter mutation), and where six mutations showed pairwise incompatibility, that is, three pairs each showed a second-order genetic interaction with fitness effect −2 (approximating the amino acid mutations), producing eight adaptive peaks. The number of potential genetic interactions to be added include 18 second order (7 × 6/2!−3 already present), 35 third order (7 × 6 × 5/3! ), 35 fourth order (7 × 6 × 5 × 4/4!) and 21 fifth order (7 × 6 × 5 × 4 × 3 /5!). Variant landscapes were generated by randomly selecting k each of the possible second-, third-, fourth- and fifth-order interactions, and assigning to each new interaction a random fitness effect between −1 and +1, such that they are no larger in magnitude than mutations’ individual effects. Two hundred such landscapes were created for each integer k . Landscapes were discarded if any new adaptive peaks were created, or if any of the eight designated adaptive peak genotypes became inaccessible from the wild-type genotype. For each landscape, all feasible evolutionary trajectories were enumerated, and the number of adaptive peaks that remain accessible at every mutational step was determined. ‘Half-commitment’ was defined as the step at which half or fewer adaptive peaks remain accessible. To calculate the average number of mutation events until half-commitment for an entire landscape, each trajectory’s ‘half-commitment’ point was weighted by the estimated probability of realization of a given trajectory, according to the equal fixation probability model (briefly, when an evolutionary trajectory has n different options for adaptive mutations, each occurs with probability n −1 ) [1] . How to cite this article : Palmer, A.C. et al . Delayed commitment to evolutionary fate in antibiotic resistance fitness landscapes. Nat. Commun. 6:7385 doi: 10.1038/ncomms8385 (2015).